Resident CD4+T cells accumulate in lymphoid organs after prolonged antigen exposure Effector and memory CD4 + T cells acquire distinct migratory properties depending on the type and location of the immune responses. Due to the highly dynamic nature of T cell circulation, the comprehensive analysis of these migratory routes requires dedicated experimental approaches. Here, we analyse the migration of effector/memory CD4 + T cells by long-term in vivo cell tracking. We identify a resident population of antigen-experienced CD4 + T cells that resides in lymph nodes and Peyer’s patches without circulation or proliferation. Resident CD4 + T cells constitute up to 50% of all effector/memory cells, including, but not limited to, follicular helper T cells. Furthermore, these non-circulating T cells possess a distinct T cell receptor repertoire and accumulate in Peyer’s patches after continuous oral antigen exposure. Our results provide the first direct evidence for a resident population of effector/memory CD4 + T cells that is retained in lymphoid tissues. Migration of CD4 + T cells is a highly coordinated process providing surveillance in lymph nodes (LNs) along with effective protection in tissues. CD62L hi naive CD4 + T cells continuously circulate through LNs searching for their cognate antigens on local antigen presenting cells. Once T cells are activated, they can fundamentally change their migratory routes as they differentiate to become antigen-experienced effector and memory cells. While most of the effector T cells down-modulate CD62L, which limits their homing to LNs, a subset of effector/memory CD4 + T cells regain CD62L expression and continues to circulate through LNs [1] , [2] , [3] . During T cell differentiation, multiple factors such as the cytokine milieu and the context of antigen presentation are integrated to arm T cells with tailored migratory and functional attributes [3] , [4] , [5] . In this respect, Peyer’s patches (PPs) represent a unique environment for CD4 + T cell responses as they are constantly exposed to microbial and antigenic stimulation from the intestine [6] . Unlike LNs, PPs constitutively comprise large germinal centres, which serve as immunoglobulin A induction sites, and follicular helper T (T FH ) cells are a major population of effector T cells in PPs. T FH cells emerged as a distinct type of effector CD4 + T cells with particular migratory properties as they express the chemokine receptor CXCR5 which allows them to migrate into B cell follicles and germinal centres [7] , [8] . In addition, T FH cells are generally regarded as LN-resident cells that stay in the LNs where they are induced. However, current information on residency of T FH cells is limited to LNs in immunized mice and mostly based on indirect evidence such as cell numbers observed under experimental blockade of egress [9] , [10] or expression levels of the egress-promoting sphingosine-1-phosphate receptor 1 ( S1pr1 ) [11] . Whether residency in LNs is an exclusive feature of T FH cells or whether there are other LN-resident effector T cell subsets remains an open question. In contrast to T cell homing, which can be studied by short-term adoptive transfer experiments, T cell residency or egress have been difficult to address due to the limitations of conventional methods. Recently, the use of photoconvertible and photoactivatable proteins provided new insights into lymphocyte trafficking [12] , [13] , [14] . These fluorescent proteins change their emission wavelength upon exposure to light of specific wavelengths. Thus, targeted illumination of cells that express such proteins allows spatiotemporal labelling of the cells. We developed two different methods by using either the photoconvertible protein Dendra2 or FITC injection to track effector/memory CD4 + T cells in LNs and PPs [15] . Here, we describe a resident population of antigen-experienced CD4 + T cells that resides in LNs and PPs for prolonged periods of time. Lymph nodes and Peyer’s patches contain resident CD4 + T cells We established a photoconversion-based cell labelling method using the photoconvertible protein Dendra2, which emits green fluorescence in its native form (D-Green), but upon illumination with UV/violet light changes into a form that emits red fluorescence (D-Red). Photoconversion of cytosolic proteins has been reported to label cells for short time periods only due to fast protein turnover rates [14] . Therefore, we used a histone (H2B)-fused version of Dendra2 that allowed us to label cells for longer time periods by increasing protein stability. To track CD4 + T cells in vivo , we prepared bone marrow (BM) chimeras using wild-type (WT) BM cells transduced with H2B-Dendra2. In these chimeras, we photoconverted the surgically exposed mesenteric lymph node (mLN), labelling all cells inside as D-Red + cells ( Fig. 1a ). After photoconversion of the mLN, D-Red + lymphocytes distributed throughout the body as naive cells continued their circulation ( Fig. 1a–d ). Seven days after photoconversion, photoconverted mLN (mLN conv ) still had the highest frequency of D-Red + cells among CD4 + T cells compared with PPs and other LNs ( Fig. 1c ). Strikingly, when we analysed CD62L lo effector/memory CD4 + T cells in mLN, 42.4±5.9% of these cells were D-Red + cells, whereas frequencies of D-Red + cells among CD62L lo CD4 + T cells in other lymphoid organs were negligible ( Fig. 1b,c ). Similarly, 7 days after photoconversion of the inguinal LN (iLN), the frequency of D-Red + cells among CD62L lo effector/memory CD4 + T cells was highest in the photoconverted iLN (iLN conv , Fig. 1e ). These results show that a significant portion of CD62L lo effector/memory CD4 + T cells are retained in LNs for at least 7 days. 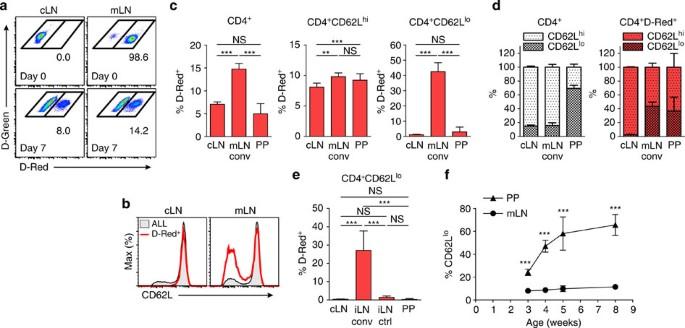Figure 1: Lymph nodes contain resident CD4+T cells. (a) Frequency of D-Red+among CD4+T cells in cervical LNs (cLN) and mLN immediately (upper panel) and 7 days (lower panel) after photoconversion of mLN (representative of three independent experiments). (b) CD62L expression on all CD4+(grey-filled histogram) and D-Red+CD4+T cells (red line) in cLN (left) and mLN (right) 7 days after photoconversion of mLN (representative of three independent experiments,n=9 mice). (c) Frequency of D-Red+among all CD4+(left), CD4+CD62Lhi(middle) and CD4+CD62Llo(right) T cells 7 days after photoconversion of mLN (n=5 mice in two independent experiments, mean±s.d., one-way analysis of variance (ANOVA), Tukey’s post test, **P<0.01; ***P<0.001; not significant (NS)). (d) Frequency of CD62Lhiand CD62Llocells among CD4+(left) or CD4+D-Red+(right) T cells 7 days after photoconversion of mLN from data inc(mean±s.d.). (e) Frequency of D-Red+among CD4+CD62LloT cells in cLN, iLNconv(photoconverted iLN), iLNctrl(non-photoconverted iLN) and PPs 7 days after photoconversion of iLN (n=4 mice in two independent experiments, mean±s.d., one-way ANOVA, Tukey’s post test, ***P<0.001; not significant (NS)). (f) Frequency of CD62Lloamong all CD4+T cells in mLN and PP of WT C57BL6/N mice at different ages (n=5–8 mice per time-point in four independent experiments, unpaired Student’st-test, ***P<0.001). Figure 1: Lymph nodes contain resident CD4 + T cells. ( a ) Frequency of D-Red + among CD4 + T cells in cervical LNs (cLN) and mLN immediately (upper panel) and 7 days (lower panel) after photoconversion of mLN (representative of three independent experiments). ( b ) CD62L expression on all CD4 + (grey-filled histogram) and D-Red + CD4 + T cells (red line) in cLN (left) and mLN (right) 7 days after photoconversion of mLN (representative of three independent experiments, n =9 mice). ( c ) Frequency of D-Red + among all CD4 + (left), CD4 + CD62L hi (middle) and CD4 + CD62L lo (right) T cells 7 days after photoconversion of mLN ( n =5 mice in two independent experiments, mean±s.d., one-way analysis of variance (ANOVA), Tukey’s post test, ** P <0.01; *** P <0.001; not significant (NS)). ( d ) Frequency of CD62L hi and CD62L lo cells among CD4 + (left) or CD4 + D-Red + (right) T cells 7 days after photoconversion of mLN from data in c (mean±s.d.). ( e ) Frequency of D-Red + among CD4 + CD62L lo T cells in cLN, iLN conv (photoconverted iLN), iLN ctrl (non-photoconverted iLN) and PPs 7 days after photoconversion of iLN ( n =4 mice in two independent experiments, mean±s.d., one-way ANOVA, Tukey’s post test, *** P <0.001; not significant (NS)). ( f ) Frequency of CD62L lo among all CD4 + T cells in mLN and PP of WT C57BL6/N mice at different ages ( n =5–8 mice per time-point in four independent experiments, unpaired Student’s t -test, *** P <0.001). Full size image In adult mice, the frequency of CD62L lo cells among all CD4 + T cells in LNs is relatively low. In contrast, this value can be as high as 70% in PPs ( Fig 1f ). Interestingly, the frequency of CD62L lo cells in PPs increases gradually with age ( Fig. 1f ). This dramatic increase was not detected in LNs; therefore, it cannot be explained solely by the overall increase in the frequency of effector/memory cells with age. Instead, changes in microbiota and diet after weaning unique to PPs might drive the accumulation of CD62L lo cells in this compartment. To investigate the circulation dynamics of effector/memory CD4 + T in PPs, we photoconverted 4–5 PPs out of the 8–10 PPs in H2B-Dendra2 BM chimeras and analysed the D-Red + cells after 7 days. Importantly, in these experiments non-illuminated PPs (PP ctrl ) served as internal controls for the circulation rates of lymphocytes as they would recruit similar cells from blood as illuminated PPs (PP conv ). Similar to mLN photoconversion, the highest frequency of D-Red + among CD4 + CD62L lo T cells was found in PP conv ( Fig. 2a ). The frequencies of D-Red + among all CD4 + T cells in other organs were much lower than the values after the photoconversion of mLN due to the comparably low number of D-Red + naive T cells introduced to the system by the photoconversion of PPs ( Fig. 2a,b ). Similar to LNs, 51.9±5.9% of CD62L lo CD4 + T cells were retained in PPs as resident cells for 7 days. Indeed, H2B-Dendra2 protein permitted the tracking lymphocytes for more than 7 days after photoconversion ( Supplementary Fig. 1 ). Although the frequency of D-Red + cells among all CD4 + T cells in PP conv remained steady for 2 weeks after photoconversion, we observed a decrease in this frequency 4 weeks after photoconversion ( Fig. 2e ). Of note, illumination of PPs did not affect viability of lymphocytes or induced stress responses ( Supplementary Fig. 2 ). 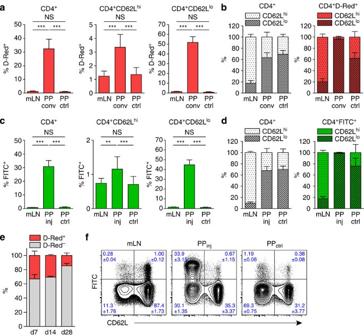Figure 2: Peyer’s patches contain resident CD4+T cells. (a) Frequency of D-Red+among all CD4+(left) ), CD4+CD62Lhi(middle) and CD4+CD62Llo(right) T cells 7 days after photoconversion of PPs (n=5 mice in three independent experiments, mean±s.d., one-way analysis of variance (ANOVA), Tukey’s post test, ***P<0.001; not significant (NS)). (b) Frequency of CD62Lhiand CD62Llocells among CD4+(left) or CD4+D-Red+(right) T cells 7 days after photoconversion of PPs from data ina(mean±s.d.). (c) Frequency of FITC+among all CD4+(left), CD4+CD62Lhi(middle) and CD4+CD62Llo(right) T cells 7 days after FITC injection into PPs (n=8 mice in two independent experiments, mean±s.d., one-way ANOVA, Tukey’s post test, **P<0.01; ***P<0.001; not significant (NS)). (d) Frequency of CD62Lhiand CD62Llocells among CD4+(left) or CD4+D-Red+(right) T cells 7 days after FITC injection into PPs from data inc(mean±s.d.). (e) Frequency of D-Red+(red bars) and D-Red−(grey bars) among CD4+T cells in PPconv7, 14 and 28 days after (n=3 mice per time-point in two independent experiments, mean±s.d.) (f) CD62L expression on CD4+T cells 7 days after FITC injection into PPs (representative of three independent experiments,n=18 mice, mean±s.d.). Figure 2: Peyer’s patches contain resident CD4 + T cells. ( a ) Frequency of D-Red + among all CD4 + (left) ), CD4 + CD62L hi (middle) and CD4 + CD62L lo (right) T cells 7 days after photoconversion of PPs ( n =5 mice in three independent experiments, mean±s.d., one-way analysis of variance (ANOVA), Tukey’s post test, *** P <0.001; not significant (NS)). ( b ) Frequency of CD62L hi and CD62L lo cells among CD4 + (left) or CD4 + D-Red + (right) T cells 7 days after photoconversion of PPs from data in a (mean±s.d.). ( c ) Frequency of FITC + among all CD4 + (left), CD4 + CD62L hi (middle) and CD4 + CD62L lo (right) T cells 7 days after FITC injection into PPs ( n =8 mice in two independent experiments, mean±s.d., one-way ANOVA, Tukey’s post test, ** P <0.01; *** P <0.001; not significant (NS)). ( d ) Frequency of CD62L hi and CD62L lo cells among CD4 + (left) or CD4 + D-Red + (right) T cells 7 days after FITC injection into PPs from data in c (mean±s.d.). ( e ) Frequency of D-Red + (red bars) and D-Red − (grey bars) among CD4 + T cells in PP conv 7, 14 and 28 days after ( n =3 mice per time-point in two independent experiments, mean±s.d.) ( f ) CD62L expression on CD4 + T cells 7 days after FITC injection into PPs (representative of three independent experiments, n =18 mice, mean±s.d.). Full size image As an alternative method to photoconversion, we used FITC injection with fine glass capillaries to label cells in PPs. After FITC injection all cells inside the injected PP (PP inj ) were labelled as FITC + cells [15] . Similar to the photoconversion method, we injected FITC into 4–5 PPs and the remaining non-injected PPs (PP ctrl ) served as internal controls. Seven days after FITC injection in WT mice, the distribution of FITC + lymphocytes was almost the same as that of D-Red + lymphocytes 7 days after photoconversion ( Fig. 2c,d,f ). In conclusion, these results clearly show that some CD4 + T cells are retained in LNs and PPs and these cells can constitute up to 50% of all CD4 + CD62L lo T cells. Of note, both D-Red and FITC signals were quickly lost from proliferating cells ( Supplementary Fig. 3a,b ), suggesting that resident CD4 + T cells are not proliferating cells within the analysed time periods. Resident CD4 + T cells are a heterogeneous population Next we analysed the resident CD4 + T cells in LNs and PPs for the expression of T FH markers PD-1 and CXCR5. In mLN, only 6.79±4.27% of the resident CD4 + CD62L lo T cells were PD-1 hi CXCR5 hi T FH cells ( Fig. 3a , Supplementary Fig. 4a ). Although PPs contain a much higher proportion of T FH cells among CD4 + T cells than mLN, PD-1 hi CXCR5 hi T FH cells represented only 20.6±2.31% of resident CD4 + CD62L lo T cells in PPs ( Fig. 3b , Supplementary Fig. 4b ). Moreover, there was only a modest enrichment of T FH cells among resident cells compared with all CD4 + T cells ( Fig. 3b ). On the other hand, in PP inj , 62.3±3.6% of PD-1 hi CXCR5 hi T FH cells were FITC + in accordance with previous reports showing most of the T FH cells to be retained in LNs ( Supplementary Fig. 5 ) [9] , [10] , [13] . 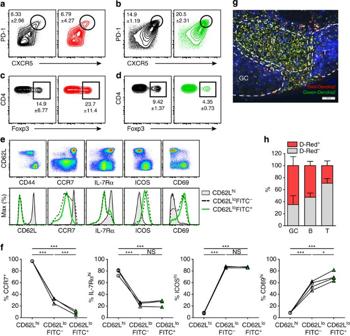Figure 3: Resident CD4+T cells are a heterogeneous population including TFHcells. (a) Frequency of PD-1hiCXCR5hiTFHcells among CD4+CD62LloT cells (left) and CD4+CD62LloD-Red+cells (right) in mLNconvafter 7 days (representative of two independent experiments,n=4 mice, mean±s.d.). (b) Frequency of PD-1hiCXCR5hiTFHcells among CD4+CD62LloT cells (left) and among CD4+CD62LloFITC+cells (right) in PPinjafter 7 days (representative of three independent experiments,n=18 mice, mean±s.d.). (c) Frequency of Foxp3+regulatory T cells for the populations as ina. (d) Frequency of Foxp3+regulatory T cells for the populations as inb. (e) Upper panels: expression of CD62L, CD44, CCR7, IL-7Rα, ICOS and CD69 on all CD4+T cells in PPinj7 days after. Lower panels: expression of CD62L, CCR7, IL-7Rα, ICOS and CD69 on CD4+CD62Lhicells (grey-filled histograms), CD4+CD62LloFITC−cells (dashed black lines) CD4+CD62LloFITC+cells (green lines) in PPinjafter 7 days (representative of at least three independent experiments). (f) Frequencies of CCR7+, IL-7Rαhi, ICOShiand CD69hicells among populations described ine(pooled samples fromn=18–24 mice in three to four independent experiments, one-way analysis of variance, Tukey’s post test, *P<0.05; ***P<0.001; not significant (NS)). (g) Histological analysis of D-Red+cells in PPconv7 days after photoconversion (GC, germinal center; B, B cell follicle; T, interfollicular T cell area, representative of two independent experiments, scale bar, 50 μm). (h) Frequency of D-Red+and D-Red−cells among all CD3+cells in different areas of PPconvas ing(six PPs from four mice in two independent experiments, mean±s.d.). Figure 3: Resident CD4 + T cells are a heterogeneous population including T FH cells. ( a ) Frequency of PD-1 hi CXCR5 hi T FH cells among CD4 + CD62L lo T cells (left) and CD4 + CD62L lo D-Red + cells (right) in mLN conv after 7 days (representative of two independent experiments, n =4 mice, mean±s.d.). ( b ) Frequency of PD-1 hi CXCR5 hi T FH cells among CD4 + CD62L lo T cells (left) and among CD4 + CD62L lo FITC + cells (right) in PP inj after 7 days (representative of three independent experiments, n =18 mice, mean±s.d.). ( c ) Frequency of Foxp3 + regulatory T cells for the populations as in a . ( d ) Frequency of Foxp3 + regulatory T cells for the populations as in b . ( e ) Upper panels: expression of CD62L, CD44, CCR7, IL-7Rα, ICOS and CD69 on all CD4 + T cells in PP inj 7 days after. Lower panels: expression of CD62L, CCR7, IL-7Rα, ICOS and CD69 on CD4 + CD62L hi cells (grey-filled histograms), CD4 + CD62L lo FITC − cells (dashed black lines) CD4 + CD62L lo FITC + cells (green lines) in PP inj after 7 days (representative of at least three independent experiments). ( f ) Frequencies of CCR7 + , IL-7Rα hi , ICOS hi and CD69 hi cells among populations described in e (pooled samples from n =18–24 mice in three to four independent experiments, one-way analysis of variance, Tukey’s post test, * P <0.05; *** P <0.001; not significant (NS)). ( g ) Histological analysis of D-Red + cells in PP conv 7 days after photoconversion (GC, germinal center; B, B cell follicle; T, interfollicular T cell area, representative of two independent experiments, scale bar, 50 μm). ( h ) Frequency of D-Red + and D-Red − cells among all CD3 + cells in different areas of PP conv as in g (six PPs from four mice in two independent experiments, mean±s.d.). Full size image Further characterization of resident CD4 + T cells revealed even more aspects of heterogeneity among these cells. In both PPs and mLN, resident CD4 + T cells included Foxp3 + regulatory T cells (Tregs). In mLN, Tregs were enriched among resident cells compared with all CD4 + CD62L lo T cells. In contrast, in PPs there were fewer Tregs among resident cells than among all CD4 + CD62L lo T cells ( Fig. 3c,d , Supplementary Fig. 4c,d ). Despite the presence of T FH and Treg cells in the resident CD4 + T cell population, resident cells in PPs shared a common phenotypic profile with regard to several other markers. Almost all resident cells were homogeneously CD62L lo , CCR7 − , ICOS hi and CD69 hi , with some cells being CD69 int/− ( Fig. 3e ). Moreover, CD62L lo FITC + resident cells contained lower frequencies of CCR7 + cells and higher frequencies of CD69 hi cells compared with CD62L lo FITC − cells ( Fig. 3f , Supplementary Fig. 6 ). Interestingly, resident CD4 + T cells in PPs contained both IL-7Rα hi and IL-7Rα lo cells indicating the presence of both memory and effector cells in this population ( Fig. 3e ). However, there was no difference between the frequencies of IL-7Rα hi cells among CD62L lo FITC + resident cells and CD62L lo FITC − cells ( Fig. 3f , Supplementary Fig. 6 ). In addition, although there was no difference between CD62L lo FITC + resident cells and CD62L lo FITC − cells in the frequencies of ICOS hi cells, resident cells expressed lower levels of ICOS ( Fig. 3e,f , Supplementary Fig. 6 ). Histological analysis of PP conv 7 days after photoconversion showed that D-Red + resident cells were present in all major compartments, that is, germinal centres, B cell follicles and interfollicular T cell areas ( Fig. 3g ). The frequency of D-Red + cells among CD3 + T cells was highest in germinal centres, in accordance with the analysis of T FH cells by flow cytometry ( Fig. 3h ). Moreover, when we analysed resident D-Red + cells in explanted PPs by two-photon microscopy, they were as motile as D-Red − cells ( Supplementary Fig. 7 ). Of note, we could not detect homing of resident CD4 + T cells to PPs or small intestinal lamina propria after adoptive transfers ( Supplementary Fig. 8 ). Resident cells have a distinct cytokine expression profile To gain insight into potential functions of resident effector/memory CD4 + T cells, we analysed the expression of different cytokines by CD62L lo FITC + resident cells and CD62L lo FITC − cells in PPs. We sorted FITC + and FITC − CD4 + CD62L lo effector/memory T cells together with CD62L hi FITC − naive CD4 + T cells from PP inj 7 days after FITC injection in WT mice. Resident cells expressed higher levels of Il4 compared with the rest of the effector/memory cells, whereas the expression of Il10 and Il17a were lower among resident cells ( Fig. 4 ). We could not detect any differences between CD62L lo FITC + resident cells and CD62L lo FITC − cells in terms of Ifng , Il21 and Tgfb1 ( Fig. 4 ). These results suggest that, in addition to their distinct migratory behaviour, effector/memory cells that are retained in PPs differ from the rest of the effector/memory cells as a population also in terms of their cytokine expression profile. Of note, we could not perform intracellular cytokine stainings on resident CD4 + T cells due to a decrease in the frequency of FITC + cells after in vitro stimulation ( Supplementary Fig. 9 ). 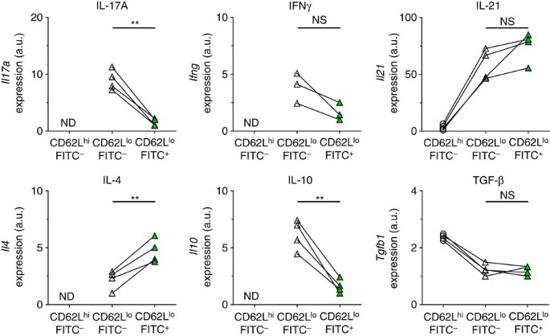Figure 4: Resident CD4+T cells have a distinct cytokine expression profile. Relative expression ofIl17a, Ifng, Il21, Il4, Il10 and Tgfb1normalized toGapdhexpression in CD62LhiFITC−, CD62LloFITC+and CD62LloFITC−CD4+T cells sorted from PPinjafter 7 days in WT mice (n=3–4 mice in two independent experiments, mean±s.d., arbitrary units (a.u.), not detected (ND), paired Student’st-test; **P<0.01, not significant (NS)). Figure 4: Resident CD4 + T cells have a distinct cytokine expression profile. Relative expression of Il17a, Ifng, Il21, Il4, Il10 and Tgfb1 normalized to Gapdh expression in CD62L hi FITC − , CD62L lo FITC + and CD62L lo FITC − CD4 + T cells sorted from PP inj after 7 days in WT mice ( n =3–4 mice in two independent experiments, mean±s.d., arbitrary units (a.u. ), not detected (ND), paired Student’s t -test; ** P <0.01, not significant (NS)). Full size image Resident cells express low levels of S1pr1 S1PR1 is the central receptor for the egress of T cells from lymphoid tissues [16] . Previous reports have shown that CD69 can bind to S1PR1 on the cell surface and block the egress of lymphocytes [17] , [18] . Moreover, retention of recently activated T cells in lymphoid organs depends on CD69 (ref. 15 ). Since most of the resident CD4 + T cells in PPs were CD69 hi , we hypothesized that CD69 might be involved in the retention of these cells in lymphoid tissues. To test this hypothesis, we generated congenically marked WT/CD69 −/− mixed H2B-Dendra2 BM chimeras and photoconverted the PPs. Seven days later, there was no significant difference in the frequency of D-Red + cells between WT and CD69 −/− CD4 + T cells in PP conv ( Fig. 5a , Supplementary Fig. 10 ). Furthermore, when we injected FITC into the PPs of CD69 −/− mice and analysed 7 days later, 24.7±10.8% of CD4 + and 48.7±8.1% of CD4 + CD62L lo cells were FITC + in PP inj which were similar to the values observed for WT mice ( Fig. 5b ). Altogether, these results indicate that CD69 is dispensable for the generation of resident CD4 + T cells in PPs. 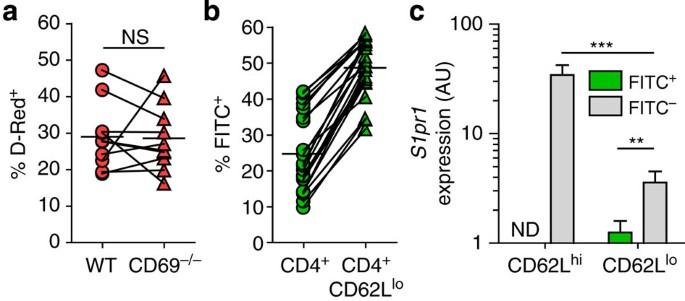Figure 5: Resident CD4+T cells express lower levels ofS1pr1than other effector/memory cells. (a) Frequency of D-Red+among WT or CD69−/−CD4+T cells in PPconv7 days after photoconversion of PPs in congenically marked WT/CD69−/−mixed Dendra2 BM chimera (n=5 mice in three independent experiments, not significant (NS,P=0.90), paired Student’st-test, line show mean value). (b) Frequency of FITC+among CD4+and CD4+CD62LloT cells in PPinjafter 7 days in CD69−/−mice. (n=6 mice in three independent experiments, lines show mean value). (c) Relative expression ofS1pr1normalized toGapdhexpression in CD62LhiFITC−, CD62LloFITC+and CD62LloFITC−CD4+T cells sorted from PPinjafter 7 days in WT mice (n=6 mice in two independent experiments, mean±s.d., arbitrary units (a.u.), not determined (ND); **P<0.01; ***P<0.001 paired Student’st-test). Figure 5: Resident CD4 + T cells express lower levels of S1pr1 than other effector/memory cells. ( a ) Frequency of D-Red + among WT or CD69 −/− CD4 + T cells in PP conv 7 days after photoconversion of PPs in congenically marked WT/CD69 −/− mixed Dendra2 BM chimera ( n =5 mice in three independent experiments, not significant (NS, P =0.90), paired Student’s t -test, line show mean value). ( b ) Frequency of FITC + among CD4 + and CD4 + CD62L lo T cells in PP inj after 7 days in CD69 −/− mice. ( n =6 mice in three independent experiments, lines show mean value). ( c ) Relative expression of S1pr1 normalized to Gapdh expression in CD62L hi FITC − , CD62L lo FITC + and CD62L lo FITC − CD4 + T cells sorted from PP inj after 7 days in WT mice ( n =6 mice in two independent experiments, mean±s.d., arbitrary units (a.u. ), not determined (ND); ** P <0.01; *** P <0.001 paired Student’s t -test). Full size image Another possible mechanism for the residency of CD4 + T cells could be the transcriptional regulation of S1pr1 . We sorted FITC + and FITC − CD4 + CD62L lo effector/memory T cells together with CD62L hi FITC − naive CD4 + T cells from PP inj 7 days after FITC injection in WT mice ( Fig. 5c ). Although both populations of CD62L lo cells expressed lower levels of S1pr1 than CD62L hi cells, CD62L lo FITC + cells expressed significantly lower levels than CD62L lo FITC − cells. This low expression of S1pr1 in resident CD4 + T cells might provide an explanation for the retention of these cells. Importantly, the FITC − fraction of CD62L lo cells contained proliferating cells, which are known to express low levels of S1pr1 (ref. 16 ). Therefore, the difference between S1pr1 expression of resident and circulating effector/memory cells might in fact be even higher than what our results suggest. Resident CD4 + T cells in PPs have a distinct TCR repertoire The observation that each PP has its own resident effector/memory CD4 + T cells implies two possible scenarios: either these cells are generated in each PP and stay in the PP that they are generated in or effector/memory CD4 + T cells seed different PPs via bloodstream and become resident after their entry into PPs. To investigate these possibilities, we injected FITC into PPs of WT mice and sorted CD62L lo FITC + and CD62L lo FITC − CD4 + T cells from individual PP inj together with CD62L lo FITC − CD4 + T cells from mLN of these mice. Then we sequenced the TCR repertoire of these different populations of CD4 + T cells focusing on Vα8 (TRAV12) family as previously described [19] . To compare the similarity between TCR repertoires, we used the Morisita–Horn index (MHI) as a measure of similarity, which takes into account both the different TCR sequences and their abundances. MHI of 1.00 indicates 100% similarity between repertoires while MHI of 0.00 means that the repertoires compared are completely dissimilar. Repertoire comparisons between CD62L lo FITC + CD4 + T cells of PPs from different mice showed MHI scores close to 0 (data not shown). In contrast, we observed considerably higher although strongly varying degrees of similarities between resident CD62L lo FITC + CD4 + T cells from different PPs in the same mouse, showing that at least some of the resident cells in different PPs share identical TCR sequences and therefore, are very unlikely to have been generated independently in different PPs ( Fig. 6a ). Instead, T cells from the circulating pools of effector/memory cells might home to PPs and after homing, some of these cells can become resident cells, while others can leave the PP and continue their circulation. However, this result does not rule out the possibility that effector/memory cells that are activated in a PP can become resident cells and stay inside that PP. Considering the intermediate values of MHI, we would suggest that generation of resident cells within the PP itself and homing of effector/memory cells from the circulation both contribute to the pool of resident cells in PPs. Moreover, the highly variable nature of similarity between the repertoires of resident cells in PPs suggests that these processes might have different contributions in different PPs. 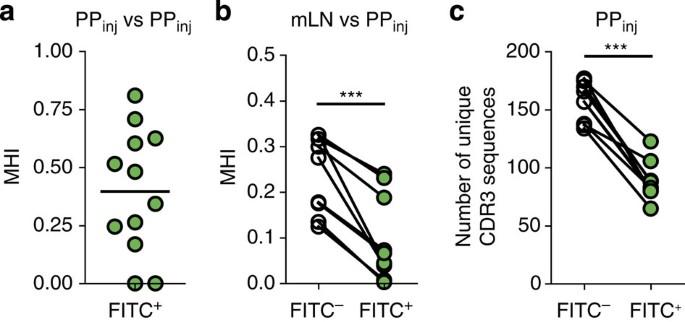Figure 6: Resident CD4+T cells have a distinct TCR repertoire. CD62LloFITC+and CD62LloFITC−CD4+T cells from PPinjtogether with CD62LloFITC−CD4+T cells from mLNs of the same mice were sorted 7 days after FITC injection into PPs of WT mice. Then TCR repertoire for Vα8 (TRAV12) family is sequenced. (15 PPs from six mice in two independent experiments). (a) Similarities between repertoires of CD4+CD62LloFITC+cells from different PPinjwithin the same mouse (MHI of 1 indicates 100% similarity). (b) The repertoires of CD4+CD62LloFITC+and CD4+CD62LloFITC−cells from PPinjwere compared with those of CD4+CD62LloFITC−cells from mLN within the same mouse and the similarities are shown as MHI (***P<0.001, paired Student’st-test). (c) Number of unique CDR3 sequences among 300 TCR sequences from FITC+and FITC−CD4+CD62Llocells from PPinj(***P<0.001, paired Student’st-test). Figure 6: Resident CD4 + T cells have a distinct TCR repertoire. CD62L lo FITC + and CD62L lo FITC − CD4 + T cells from PP inj together with CD62L lo FITC − CD4 + T cells from mLNs of the same mice were sorted 7 days after FITC injection into PPs of WT mice. Then TCR repertoire for Vα8 (TRAV12) family is sequenced. (15 PPs from six mice in two independent experiments). ( a ) Similarities between repertoires of CD4 + CD62L lo FITC + cells from different PP inj within the same mouse (MHI of 1 indicates 100% similarity). ( b ) The repertoires of CD4 + CD62L lo FITC + and CD4 + CD62L lo FITC − cells from PP inj were compared with those of CD4 + CD62L lo FITC − cells from mLN within the same mouse and the similarities are shown as MHI (*** P <0.001, paired Student’s t -test). ( c ) Number of unique CDR3 sequences among 300 TCR sequences from FITC + and FITC − CD4 + CD62L lo cells from PP inj (*** P <0.001, paired Student’s t -test). Full size image When we compared the TCR repertoires of FITC + and FITC − populations of effector/memory cells from PP inj to effector/memory cells from mLN, FITC + resident PP cells were less similar to mLN than were the rest of the effector/memory cells in PP inj ( Fig. 6b ). In addition, resident cells had a significantly lower TCR repertoire diversity than the remainder of the effector/memory population in the same PP inj , as shown by the lower number of unique complementary determining region 3 (CDR3) sequences ( Fig. 6c ). Altogether, these results suggest that CD4 + T cells retained in PPs have different TCR repertoires than other effector/memory cells, which implies clonal history and/or TCR signalling to be important factors in the generation of resident CD4 + T cells. CD4 + T cells with diverse TCR sequences accumulate in PPs To investigate the involvement of TCR signalling in the induction of resident cells, we analysed RAG-sufficient OT-II transgenic mice in which most CD4 + T cells express the OT-II TCR composed of Vα2 and Vβ5 chains specific for an ovalbumin (OVA) peptide. However, in these mice there are still CD4 + T cells that express diverse TCRs resulting from endogenous recombination events. Although these CD4 + T cells that do not express the OT-II TCR (Vβ5 − ) were relatively few in LNs, they comprised 42.1±9.9% of all CD4 + T cells in PPs ( Fig. 7a , Supplementary Fig. 11a ). Furthermore, almost all of these Vβ5 − CD4 + T cells in PPs were CD62L lo , indicating an antigen-experienced phenotype ( Fig. 7b,c , Supplementary Fig. 11b ). To address whether there are resident cells among these Vβ5 − CD4 + T cells, we injected FITC into the PPs of OT-II mice and analysed them 7 days later. Consistent with their naive phenotype, very few FITC + Vβ5 + cells were present in PP inj 7 days after FITC injection. In contrast, 44.7±12.8% of Vβ5 − CD4 + T cells were FITC + in PP inj indicating the presence of resident cells in this population ( Fig. 7c ). These results further support the notion that some antigen-experienced CD4 + T are retained in PPs as resident cells. 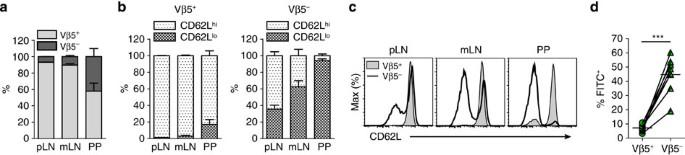Figure 7: Vβ5−CD4+T cells accumulate as resident cells in PPs of RAG-sufficient OT-II mice. (a) Frequency of TCR Vβ5+(dark-grey bars) and Vβ5−(light-grey bars) cells among CD4+T cells in non-manipulated RAG-sufficient OT-II mice. (n=5 mice in two independent experiments, peripheral LN (pLN), mean±s.d.) (b) Frequency of CD62Lhiand CD62Llocells among Vβ5+(left) and Vβ5−(right) CD4+T cells froma(mean±s.d.). (c) CD62L expression on Vβ5+and Vβ5−CD4+T cells froma(representative of three independent experiments). (d) Frequency of FITC+cells among Vβ5+and Vβ5−CD4+cells in PPinjafter 7 days in OT-II mice (n=4 mice in two independent experiments; ***P<0.001, paired Student’st-test, lines show mean value). Figure 7: Vβ5 − CD4 + T cells accumulate as resident cells in PPs of RAG-sufficient OT-II mice. ( a ) Frequency of TCR Vβ5 + (dark-grey bars) and Vβ5 − (light-grey bars) cells among CD4 + T cells in non-manipulated RAG-sufficient OT-II mice. ( n =5 mice in two independent experiments, peripheral LN (pLN), mean±s.d.) ( b ) Frequency of CD62L hi and CD62L lo cells among Vβ5 + (left) and Vβ5 − (right) CD4 + T cells from a (mean±s.d.). ( c ) CD62L expression on Vβ5 + and Vβ5 − CD4 + T cells from a (representative of three independent experiments). ( d ) Frequency of FITC + cells among Vβ5 + and Vβ5 − CD4 + cells in PP inj after 7 days in OT-II mice ( n =4 mice in two independent experiments; *** P <0.001, paired Student’s t -test, lines show mean value). Full size image Continuous antigen supply results in accumulation of effector cells in PPs Both TCR repertoire analysis and results from TCR-transgenic OT-II mice suggested TCR signalling and antigen presentation to be important aspects in the generation of resident cells in lymphoid tissues. Therefore, we tried to generate resident OT-II cells in PPs by providing the cognate antigen OVA. After adoptive transfer of congenically marked (CD45.1 + ) OT-II cells, we immunized WT mice orally with OVA+cholera toxin (CT, Fig. 8a ). Seven days after immunization, CD4 + CD45.1 + Vβ5 + CD62L lo effector OT-II cells were present in both mLN and PPs ( Fig. 8b,c ). When we provided OVA in the drinking water after immunization, the frequency of CD45.1 + Vβ5 + CD62L lo among CD4 + T cells increased dramatically in PPs with a nonsignificant decrease in mLN ( Fig. 8b,c ). To assess whether these cells are retained in PPs we performed FITC injection into PPs on day 14 after immunization and analysed on day 21 by providing the antigen continuously (day 0–21) or for the first week only (day 0–7) in the drinking water ( Fig. 8d ). Surprisingly, the majority of effector OT-II cells were FITC + in PP inj in both continuous and first-week-only OVA treatment groups although there were significantly more effector OT-II cells when the antigen was supplied continuously ( Fig. 8e–g ). In addition, resident OT-II cells contained both PD-1 hi CXCR5 hi T FH and Foxp3 + Treg cells ( Supplementary Fig. 12 ). Although the frequencies of Treg cells were relatively low, both continuous and first-week-only antigen treatments induced similar frequencies of T FH and Treg cells among resident OT-II cells in PPs ( Supplementary Fig. 12 ). These results indicate that prolonged antigen supply can cause accumulation of effector cells in PPs and most of these cells were retained in PPs as resident cells. 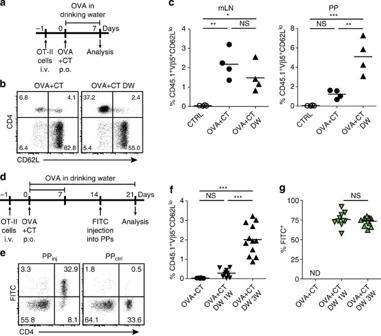Figure 8: Continuous antigen supply generates resident CD4+T cells in PPs. (a) Experimental setup for (b,c), wherein 2 × 107CD45.1+spleen/LNs cells from OT-II mice were adoptively transferred into WT recipients. One day later, some of the mice were immunized with 50 mg OVA+10 μg CT p.o. (OVA+CT) or not (CTRL). Then some of the immunized mice received OVA in drinking water for 1 week (OVA+CT DW). (b) CD45.1+transferred cells in PPs 7 days after immunization (representative of three independent experiments). (c) Frequency of CD45.1+Vβ5+CD62Lloamong all CD4+T cells in mLN (left) and in PPs (right) (n=4 mice per group in three independent experiments, not significant (NS); *P<0.05; **P<0.01; ***P<0.001; one-way analysis of variance (ANOVA), Tukey’s post test). (d) Experimental setup fore–g, wherein 14 days after immunization, FITC was injected into the PPs and mice were analysed 7 days later (day 21). Mice received OVA in the drinking water for 1 week (days 0–7, OVA+CT DW 1W) or for 3 weeks (d0–21, OVA+CT DW 3W), or not (OVA+CT). (e) CD45.1+transferred cells in PPinj(left) and PPctrl(right) in a mouse from OVA+CT DW 3W group (representative of two independent experiments). (f) Frequency of CD45.1+Vβ5+CD62Lloamong all CD4+cells in PPinj(n=3–5 mice per group in two independent experiments not significant (NS); ***P<0.001; one-way ANOVA, Tukey’s post test). (g) Frequency of FITC+among CD4+CD45.1+Vβ5+CD62Llocells in PPinj(Not determined (ND), not significant (NS), unpaired Student’st-test). i.v., intravenous. Figure 8: Continuous antigen supply generates resident CD4 + T cells in PPs. ( a ) Experimental setup for ( b , c ), wherein 2 × 10 7 CD45.1 + spleen/LNs cells from OT-II mice were adoptively transferred into WT recipients. One day later, some of the mice were immunized with 50 mg OVA+10 μg CT p.o. (OVA+CT) or not (CTRL). Then some of the immunized mice received OVA in drinking water for 1 week (OVA+CT DW). ( b ) CD45.1 + transferred cells in PPs 7 days after immunization (representative of three independent experiments). ( c ) Frequency of CD45.1 + Vβ5 + CD62L lo among all CD4 + T cells in mLN (left) and in PPs (right) ( n =4 mice per group in three independent experiments, not significant (NS); * P <0.05; ** P <0.01; *** P <0.001; one-way analysis of variance (ANOVA), Tukey’s post test). ( d ) Experimental setup for e – g , wherein 14 days after immunization, FITC was injected into the PPs and mice were analysed 7 days later (day 21). Mice received OVA in the drinking water for 1 week (days 0–7, OVA+CT DW 1W) or for 3 weeks (d0–21, OVA+CT DW 3W), or not (OVA+CT). ( e ) CD45.1 + transferred cells in PP inj (left) and PP ctrl (right) in a mouse from OVA+CT DW 3W group (representative of two independent experiments). ( f ) Frequency of CD45.1 + Vβ5 + CD62L lo among all CD4 + cells in PP inj ( n =3–5 mice per group in two independent experiments not significant (NS); *** P <0.001; one-way ANOVA, Tukey’s post test). ( g ) Frequency of FITC + among CD4 + CD45.1 + Vβ5 + CD62L lo cells in PP inj (Not determined (ND), not significant (NS), unpaired Student’s t -test). i.v., intravenous. Full size image The migratory routes of memory T cells have been broadly classified into two categories, effector memory (T EM ) and central memory (T CM ) T cells [3] , [4] . T EM cells are CD62L lo CCR7 − cells and preferentially home to non-lymphoid tissues while T CM cells are CD62L hi CCR7 + and circulate through lymphoid tissues. Together with non-lymphoid tissue resident memory T (T RM ) cells, T EM and T CM cells have been presumed to represent the main migratory specializations of effector and memory T cells. Lymphoid-tissue resident CD4 + T cells described here provide the first direct evidence for an additional migratory specialization for antigen-experienced CD4 + T cells. Indeed, we observed that up to 50% of all CD62L lo effector/memory CD4 + T cells were retained in lymphoid organs for several weeks. For technical reasons, we could not follow the fate of these cells for longer than 4 weeks (see below). Still, for the purpose of this study, we refer to these cells as lymphoid tissue ‘resident’ cells to describe their non-circulating phenotype. We propose that effector/memory CD4 + T cells can also become resident cells in lymphoid tissues in addition to previously described migratory routes. Long-term analysis of lymphocyte circulation has been challenging due to the lack of suitable methods. Therefore, detection of resident cells in lymphoid organs required dedicated experimental approaches. Photoconvertible and photoactivatable proteins considerably advanced our tool box to study cell migration and have been used previously for cell tracking in LNs and PPs [12] , [13] , [14] . Yet, these reports analysed cell migration for hours or few days only. Using a histone-fused photoconvertible protein, we managed to extend the possible period of analysis up to weeks ( Supplementary Fig. 1 ). Histone proteins are stable proteins with half-lives in the range of 3–6 months [20] , [21] . We were able to track nonproliferating lymphocytes for more than 4 weeks after photoconversion. However, we observed a reduction in the D-Red signal of the D-Red + lymphocytes 4 weeks after photoconversion ( Supplementary Fig. 1 ). This suggests that although we substantially increased the stability of the photoconverted Dendra2 protein by fusing it with a histone protein, H2B-Dendra2 protein was less stable than a native histone H2B protein. We detected a decrease in the frequency of D-Red + cells among CD4 + T cells 4 weeks after the photoconversion. At present, we cannot know the reason for the decrease in frequency of D-Red + cells. Egress, proliferation or death of the resident CD4 + T cells over time can all result in this decrease in the frequency of D-Red + cells and have to be considered beside a decline in D-Red signal due to protein turnover alone. Here we used two different methods of long-term in vivo lymphocyte tracking to analyse circulation dynamics of CD4 + T cells in different lymphoid organs. This approach requires analysis of lymphocyte circulation from a broad systemic perspective as in situ labelling of lymphocytes will generate different circulating populations of labelled cells for different lymphoid organs. For example, photoconversion of PPs will generate relatively low numbers of D-Red + CD62L hi naive T cells compared with photoconversion of mLN, due to the different cellular composition and cell numbers of PPs and mLN. Therefore, the frequencies of D-Red + naive T cells in non-photoconverted lymphoid organs will be different in these cases. Moreover, comparison of photoconverted and non-photoconverted lymphoid organs is also crucial for the accurate characterization of migratory properties of lymphocytes. For example, we identified D-Red + CD4 + CD62L lo cells in PP conv as resident cells by considering the negligible frequency of D-Red + CD4 + CD62L lo cells homing to PP conv from the circulation which was estimated by analysing PP ctrl . The migratory behaviour of resident CD4 + T cells described herein differs from the well-known antigen-specific sequestration of activated T cells in LNs carrying that antigen [22] , [23] . In these cases, responding T cells have been reported to re-enter the circulation 3 days after antigen recognition. Therefore, the residence of antigen-experienced CD4 + T cells in lymphoid tissues cannot be explained by this phenomenon. In addition, proliferating T cells in the initial phases of an immune response cannot account for this non-circulating population of CD4 + T cells because proliferating cells rapidly lose the D-Red or FITC signals ( Supplementary Fig. 2 ). CD69 upregulation is usually considered as a marker for the activation of T cells by TCR engagement or cytokine stimulation [24] . Due to its interaction with S1PR1 on the cell surface, CD69 has been assumed to have an important role in the long-term residence of T RM cells in non-lymphoid tissues as most of these cells have a CD69 hi surface phenotype [2] . In a recent study, transcriptional downregulation of S1pr1 has been suggested to be an essential part of the development of CD8 + T RM cells [25] . This transcriptional downregulation has been shown to be responsible in most cases for their CD69 hi surface phenotype and residence in non-lymphoid tissues. Consistently, in our study, resident CD4 + T cells in lymphoid tissues expressed low levels of S1pr1 and their generation was independent of CD69. Therefore, we speculate that antigen-experienced CD4 + T cells that are retained in lymphoid tissues described herein might share retention mechanisms with T RM cells. T FH cells perform their functions in lymphoid organs and previous reports have suggested T FH cells to stay in draining LNs as effector and memory cells [9] , [10] . In these studies, retention of T FH cells has been compared with the retention of other effector T cell populations after systemic blockade of lymphocyte egress. However, this approach could not detect other types of LN-resident CD4 + T cells or provide an estimate on the proportion of T FH cells that remained in LNs. Another study has also shown the majority of T FH cells to stay in the LNs for 36 h by using a photoactivation method [13] . Our results are in aggreement with these observations providing direct evidence for long-term residence of T FH and importantly reveal that long-term residency in LNs and PPs is not an exclusive feature of T FH cells. In LNs, resident T FH cells have been suggested to possess a more restricted TCR repertoire with higher affinities than the rest of the helper T cell population [10] . Although we did not focus our analysis on T FH cells, our results are in accordance with this observation, as resident CD4 + T cells in PPs possessed a less diverse TCR repertoire than the rest of the effector/memory population. TCR repertoire of resident cells in PPs was different from the repertoire of the rest of the effector/memory cells in terms of both diversity and similarity to effector/memory cells in mLN. This distinct TCR repertoire of resident cells suggests specific retention of certain T cells in lymphoid tissues rather than nonspecific slow egress of all antigen-experienced CD4 + T cells. Using OVA-specific OT-II T cells, we identified prolonged oral antigen exposure to be necessary for the accumulation of resident cells in PPs. Interestingly, even after only 1 week of continuous antigen application, the frequency of resident cells among effector OT-II cells in PPs was as high as seen after 3 weeks of antigen treatment. As we did not observe an accumulation of effector cells in PPs without continuous antigen treatment, we speculate that a brief period of continuous antigen exposure is decisive for the generation of resident antigen-experienced CD4 + T cells in PPs. Together with the distinct TCR repertoire of resident cells, these results suggest antigen presentation and TCR signalling to be important aspects of resident CD4 + T cell induction. Although we observed that antigen-experienced CD4 + T cells were retained in both LNs and PPs, the compositions of functional T cell subsets contributing to these resident cells differed between various lymphoid tissues. Moreover, prolonged antigen exposure induced the specific accumulation of resident CD4 + T cells in PPs but not in the gut-draining mLN. Since multiple cytokines as well as TCR signalling are reported to downregulate S1pr1 expression [16] , [26] , it is possible that distinct microenvironments might retain CD4 + T cells in distinct lymphoid tissues. Here we describe a population of antigen-experienced CD4 + T cells with a distinct migratory phenotype. However, it is not yet clear whether there are also functional differences between resident cells and the rest of the effector/memory cells in lymphoid organs in addition to their differences in migratory properties. Although a distinct cytokine expression profile of resident cells suggests functional differences, it is difficult to define a general functional role for resident cells due to the heterogeneous nature of this population. It is reasonable to assume that each distinct functional subset among resident cells can perform different functions, despite having the same migratory phenotype. In conclusion, our results reveal a previously unappreciated aspect of effector and memory CD4 + T cell distribution throughout the body that might provide new insights for the development of more effective vaccines. Strategic positioning of T RM cells at pathogen entry sites increases their chances to re-encounter the pathogen that originally induced their generation. Thus, T RM cells are thought to provide an advantage for early control of secondary infections [1] , [2] , [3] . Retention of effector and memory cells in a responding lymphoid tissue might serve a similar function and increase the efficacy of a secondary response to recurrent infections via the same entry route. Mice WT C57BL/6N (Charles River, Sulzfeld, Germany), CD45.1 + (B6.SJL-PtprcaPepcb/BoyJ), μMT −/− (B6.129S2-Ighmtm1Cgn/J), OT-II CD45.1 + (B6.Cg-Tg(TcraTcrb)425Cbn/J × B6.SJL-PtprcaPepcb/BoyJ) and CD69 −/− (B6.129P2-Cd69tm1Naka) were bred and reared at the Central Animal Facility of Hannover Medical School under specified pathogen-free conditions. Gender- and age-matched mice were used in all experiments for all groups. For BM chimeras, 6–8 weeks old mice were used for irradiation and these mice were used in experiments at least 6 weeks after irradiation. In other experiments, 6–12 weeks old mice were used. All experiments were approved by Lower Saxony State Office for Consumer Protection and Food Safety (Landesamt für Verbraucherschutz und Lebensmittelsicherheit, LAVES) and performed in accordance with the relevant local guidelines and regulations. All experiments were performed in compliance with ethical regulations of German Law for the Protection of Animal Welfare (Tierschutzgesetz). Flow cytometry Single-cell suspensions were prepared by meshing LNs, PPs and spleens through nylon filters in phosphate-buffered saline solution containing 3% fetal calf serum (PBS/FCS). Subsequent steps of surface stainings also performed in PBS/FCS. Blocking was performed with PBS/FCS solution containing 5% rat serum. Appropriate combinations of monoclonal antibodies CD4 (RM4-5, BioLegend, 1:400), CD8α (53-6.7, BioLegend, 1:400), CD19 (6D5, BioLegend, 1:400), CD62L (MEL-14, BioLegend, 1:200), CD44 (IM7, BioLegend, 1:200), CD45.1 (A20, BioLegend, 1:200), CD45.2 (104, BioLegend, 1:200), PD-1 (J43, eBiosciences, 1:200), CXCR5 (2G8, BD, 1:50), Foxp3 (FJK-16s, eBiosciences, 1:200), CCR7 (4B12, eBiosciences, 1:10), IL-7Rα (A7R34, BioLegend, 1:40), ICOS (C398.4A, BioLegend, 1:200), CD69 (H1.2F3, BioLegend, 1:200) and TCR-Vβ5 (MR9-4, BD, 1:400) were used for stainings. For Foxp3 stainings, Foxp3 staining kit from eBiosciences was used according to manufacturer’s instructions. All measurements were done on LSR II (BD) and analysed using FlowJo software (Tree Star). BM chimeras To generate H2B-Dendra2-expressing virus particles, MigH2BD2 (ref. 15 ) and pCL-Eco plasmids were transfected into HEK-293T cells using a calcium phosphate transfection kit (Invitrogen) and virus-containing supernatants were harvested. BM precursor cells were enriched by depleting lineage-committed cells using an antibody cocktail (CD11b, CD8β, CD49b, CD4, Gr-1, B220, CD11c and CD19) and Dynabeads (Invitrogen). Enriched BM precursor cells were cultured with IL-7 (25 ng ml −1 ), IL-6 (20 ng ml −1 ), SCF (50 ng ml −1 ) and Flt3L (23 ng ml −1 ) for 4 days and transduced with H2B-Dendra2-expressing viruses on day 2 and 4 using spin infection. On day 5, cells were harvested and 10 6 cells per recipient were transferred intravenously to lethally irradiated (10 Gy) recipients. Mice were given antibiotics (Cotrimoxazol, Ratiopharm Ulm, Ulm, Germany) in the drinking water (0.96 mg ml −1 ) for 2 weeks and analysed after 6 weeks or later. Photoconversion and FITC injection Mice were anaesthetized using ketamine and xylazine. The small intestine and caecum were exposed through a small midline incision into the skin and the abdominal wall for surgeries involving mLN and PPs. For photoconversion of iLN, the right iLN was exposed through a small incision into the skin. After surgery, all the wounds were closed with suture. For photoconversion of mLN, iLN or PPs, target tissues were illuminated for 20 s (for mLN and iLN) or 10 s (for PPs) at a low intensity light from a BlueWave 75 light curing system (Dymax, Torrington, CT) equipped with a 390/40 band pass filter with an intensity of 120 mW cm −2 . The output light was not collimated. The distance between the tip of the light source and the tissue was 1 cm and the illumination area at the target tissue was a circle with a diameter of approximately 1 cm. During illumination, tissue surrounding the mLN, iLN or PPs was covered with aluminium foil to avoid unwanted photoconversion. For photoconversion of PPs, four to five Peyer’s patches were photoconverted per mouse and their positions were mapped for analysis. For FITC injections into PPs, four to five PPs per mouse were injected with FITC (Sigma-Aldrich) (1 mg ml −1 in PBS) using custom-made glass capillaries mounted to a micro-injector (Harvard Apparatus, MA, USA). Histology Seven days after photoconversion, illuminated PPs were excised from the small intestine and frozen in Tissue-Tek O.C.T. (Fischer Scientific). Then 8 μm sections were prepared from these PPs and fixed with ice-cold acetone and stored at −20 °C. For staining, sections were rehydrated in TBST buffer (Tris-buffered saline plus Tween-20). Then, sections were blocked with 5% rat serum in TBST and stained with CD3-AlexaFluor 647 antibody for 1 h. After the staining, sections were washed with TBST and mounted with Mowiol. For the analysis of the images, PPs were divided into three areas as germinal centre, B cell follicle and interfollicular T cell areas considering the overall cell density and density of CD3 + T cells. Cell sorting DAPI − CD19 − CD8 − CD4 + lymphocytes were sorted for populations specified in the main text using XDP cell sorter (Beckman Coulter). For real-time PCR experiments, PP inj s from each mouse were pooled whereas for TCR sequencing experiments each PP inj are sorted individually. Real-time PCR RNA isolation from sorted populations was performed with RNeasy Micro kit (QIAGEN) followed by cDNA synthesis with SuperScript III Reverse Transcriptase using random hexamer primers. Real-time PCR was performed using a Light Cycler 2.0 System (Roche) and SYBR Green detection (Takara) with primers; S1pr1 -forward 5′- GGAGGTTAAAGCTCTCCGC -3′, S1pr1 -reverse 5′- CGCCCCGATGTTCAAC -3′, Gapdh -forward 5′- GTGCCAGCCTCGTCCCGTAG -3′, Gapdh -reverse 5′- TTGCCGTGAGTGGAGTCATAC -3′, Il10 -forward 5′- TGGCCCAGAAATCAAGGAGC -3′, Il10 -reverse 5′- TGGCCTTGTAGACACCTTGG -3′, Ifng -forward 5′- GACAATCAGGCCATCAGCAAC -3′, Ifng -reverse 5′- GGATGAGCTCATTGAATGCTTGG -3′, Il4 -forward 5′- GAAGAACTCTAGTGTTCTCATGG -3′, Il4 -reverse 5′- CAGGAAGTCTTTCAGTGATGTGG -3′, Il21 -forward 5′- GACATTCATCATTGACCTCGTG -3′, Il21 -reverse 5′- TCACAGGAAGGGCATTTAGC -3′, I l17a -forward 5′- AAGGCAGCAGCGATCATCC -3′, Il17a -reverse 5′- GGAACGGTTGAGGTAGTCTGAG -3′, Tgfb1 -forward 5′- TGGAGCAACATGTGGAACTC -3′, Tgfb1 -reverse 5′- CAGCAGCCGGTTACCAAG -3′. All expression levels were normalized to Gapdh expression and relative expression levels were determined using 2 −ΔΔCt method. TCR sequencing and analysis TCR repertoire sequencing was performed as previously described [19] . RNA isolation from sorted populations was performed with RNeasy Micro kit (Qiagen) followed by cDNA synthesis with SuperScript III Reverse Transcriptase using random hexamer primers. TCR sequences containing the CDR3 regions for Vα8 (TRAV12) family were amplified by PCR using primers 5′- CGTATCGCCTCCCTCGCGCCATCAGCCTTCCATCTGCAGAAGTCC -3′ and 5′- CTATGCGCCTTGCCAGCCCGCTCAG -[MID]- AGAGGGTGCTGTCCTGAGAC -3′ in which [MID] represents the multiplex identifier sequence specific for each sample. Amplicons were purified by agarose gel electrophoresis and QIAquick Gel Extraction kit (Qiagen). Then, amplicons were sequenced with 454 pyrosequencing technique (Roche). TCR sequences were analysed according to the International ImMunoGeneTics Information System (IMGT) database and only productive TCR sequences were used for further analysis. TCR repertoires were compared using MHI, which takes into account not only sequence similarities but also frequency distributions of the sequences. MHI of 1 indicates 100% similarity. Cell transfers and immunizations A total of 2 × 10 7 OT-II CD45.1 + cells from spleen and LNs were transferred intravenously into WT recipients. For immunizations, mice received p.o. 50 mg OVA (Sigma-Aldrich, grade III) together with 10 μg cholera toxin (Sigma-Aldrich) per mouse. Then 10 mg ml −1 OVA in drinking water was given for the groups indicated in the main text. Statistics Statistical analysis was performed using GraphPad Prism software. For comparison of unmatched two groups unpaired Student’s t -test was used. For comparison of matched samples (for example, values from the same PP) paired Student’s t -test was used. For comparison between three or more groups, one-way analysis of variance followed by Tukey’s post test was used unless otherwise specified in the figure legend. All data are presented as mean±s.d. and P <0.05 are considered as significant. In all figures, * P <0.05; ** P <0.01; *** P <0.001; NS, not significant. How to cite this article: Ugur, M. et al . Resident CD4 + T cells accumulate in lymphoid organs after prolonged antigen exposure. Nat. Commun. 5:4821 doi: 10.1038/ncomms5821 (2014).